A nanocomposite superstructure of metal oxides with effective charge transfer interfaces The alignment of nanoparticle building blocks into ordered superstructures is one of the key topics in modern colloid and material chemistry. Metal oxide mesocrystals are superstructures of assembled nanoparticles of metal oxides and have potentially tunable electronic, optical and magnetic properties, which would be useful for applications ranging from catalysis to optoelectronics. Here we report a facile and general approach for synthesizing metal oxide mesocrystals and developing them into new nanocomposite materials containing two different metals. The surface and internal structures of the mesocrystals were fully characterized by electron microscopy techniques. Single-particle confocal fluorescence spectroscopy, electron paramagnetic resonance spectroscopy and time-resolved diffuse reflectance spectroscopy measurements revealed that efficient charge transfer occurred between n -type and p -type semiconductor nanoparticles in the composite mesocrystals. This behaviour is desirable for their applications ranging from catalysis, optoelectronics and sensing, to energy storage and conversion. The concept of a mesocrystal, which is defined as the ordered aggregation of crystalline nanoparticles into an ordered superstructure on the scale of several hundred nanometres to micrometres, was first proposed by Cölfen and Antonietti in 2005 (refs 1 , 2 , 3 , 4 ). This definition has developed in the years, where mesocrystals are defined entirely according to their structures and not according to their formation mechanism [5] . So far, a variety of mesocrystals of metal oxides (for example, TiO 2 , ZnO, Fe 2 O 3 and CuO) have been synthesized [6] , [7] , [8] , [9] , [10] . The method most commonly used to synthesize mesocrystal materials is based on hydrothermal/solvothermal treatments [11] , [12] , [13] , [14] , in which the solution should be maintained at a specific temperature and aged for a specific period of time. The resulting precipitates are then collected and washed to remove impurities, and, in some cases, the precipitates also require further annealing. In recent years, new methods such as microwave-assisted hydrothermal [15] , bioinspired [16] and titration [17] methods have been developed to simplify the synthesis procedure and improve its efficiency. For instance, Zhou et al. [6] prepared anatase TiO 2 mesocrystals by topotactically transforming NH 4 TiOF 3 crystals without changing their morphology. Our group has recently demonstrated that anatase TiO 2 mesocrystals can be synthesized via topotactic transformation using one-step direct annealing of a titanium solution as a precursor [7] . Since these synthesis conditions are optimized for the production of the desired materials, however, a facile and general approach to the synthesis of mesocrystals of various metal oxides has not been established yet. This lack of a general approach limits the development of the mesocrystals and leads to difficulty in producing nanocomposite mesocrystals, in which two or more different types of metal oxide nanoparticles are assembled into a single mesocrystal. Such composite materials are important materials for a wide range of applications [18] , [19] , [20] , since they not only combine the properties of the building blocks but also provide new properties emerging from interfacial interactions and reactions between the different materials. On-demand engineering of self-assembled materials with highly ordered structures thus allows us to tune the electronic, optical and magnetic properties, which should provide superior performance in various applications including catalysis, sensing, (magneto)optoelectronics and solar energy conversion [21] , [22] . Herein we describe a significantly improved method of synthesizing metal oxide mesocrystals using one-step direct annealing of aqueous precursor solutions containing metal ions (M + ), NH 4 NO 3 and the amphiphilic triblock copolymer polyethylene oxide/poly( p -phenylene oxide)/polyethylene oxide (P123). As the annealing temperature is increased, the M + and NH 4 NO 3 begin a series of combination reactions, and P123 assists in assembling the nanoparticles into intermediate crystals, followed by topotactic transformation from intermediate crystals to mesocrystals. The most remarkable advantage of this method is that it can produce several mesocrystals under the same synthesis conditions, which ensures the development of new nanocomposite mesocrystal materials for efficient charge separation. To the best of our knowledge, this is the first example of the successful synthesis of such mesocrystals. 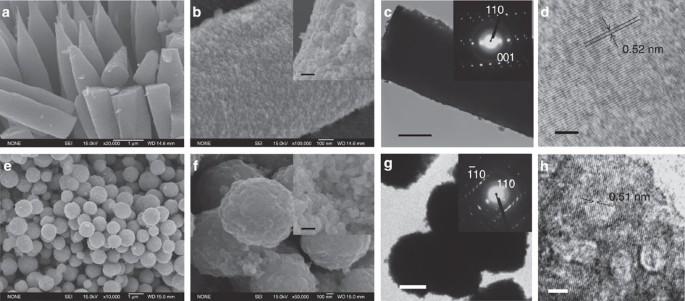Figure 1: Pure metal oxide mesocrystals. (a,b) FESEM images of ZnO. Inset of the panelcshows the interior particles at the broken part. Scale bars, 1 μm and 100 nm;aandb, respectively. (c) TEM image of ZnO. Scale bar, 500 nm. (d) HRTEM image of ZnO. Scale bar, 5 nm. (e,f) FESEM image of CuO. Inset of the panelfshows the interior particles at the broken part. Scale bars, 1 μm and 100 nm;eandf, respectively. (g) TEM image of CuO. Scale bar, 500 nm. (h) HRTEM image of CuO. Scale bar, 5 nm. SAED patterns (insets of TEM images) show the single-crystal diffraction. Structure of metal oxide mesocrystals Figure 1 shows field-emission scanning electron microscopy (FESEM) and transmission electron microscopy (TEM) images of the as-synthesized ZnO mesocrystals. The ZnO mesocrystals have rod-like structures that are ~1 μm wide and several micrometres long ( Fig. 1a,b ) and are assembled from small nanoparticles, as confirmed by FESEM images of the broken part (inset of Fig. 1b ). The selected-area electron diffraction (SAED) pattern recorded for an individual ZnO rod (inset of Fig. 1c ) reveals that the products have a single-crystalline structure, which is consistent with crystallographically oriented aggregation between primary ZnO nanocrystals. High-resolution TEM (HRTEM) images taken from the (001) planes show a hexagonal Wurtzite-type crystal with a lattice spacing of 0.52 nm ( Fig. 1d ). Figure 1f–h shows FESEM and TEM images of the CuO mesocrystals. The CuO mesocrystals are sphere like with sizes of around 500 nm in diameter ( Fig. 1e ). High-magnification FESEM and SAED images reveal perfectly oriented aggregation between the primary metal oxide nanocrystals ( Fig. 1f,g ). HRTEM images taken from the CuO mesocrystals further reveal crystalline lattice spacings of around 0.51 nm ( Fig. 1h ). Other metal oxide mesocrystals such as TiO 2 and NiO were also successfully synthesized under the same conditions ( Supplementary Fig. 1 ). Nitrogen sorption experiments indicated that the mesocrystals have mesoporous structures ( Supplementary Fig. 2 ), and the surface areas of the ZnO and CuO mesocrystals were found to be around 0.8 and 2.2 m 2 g −1 , respectively ( Supplementary Table 1 ), which are similar to reported values [23] , [24] . Although ZnO nanocrystals with sizes of >40 nm are known to have low surface areas (<10 m 2 g −1 ) [25] , [26] , the partial crystallographic fusion of adjacent faces during the calcination process may further reduce the surface area of the mesocrystals. Control experiments verified that the presence of both P123 and NH 4 NO 3 is critical for the production of mesocrystals. As shown in Supplementary Figs 3 and 4 , no mesocrystals were formed in the absence of either P123 or NH 4 NO 3 , and only macroaggregates or irregularly shaped particles were obtained. Figure 1: Pure metal oxide mesocrystals. ( a , b ) FESEM images of ZnO. Inset of the panel c shows the interior particles at the broken part. Scale bars, 1 μm and 100 nm; a and b , respectively. ( c ) TEM image of ZnO. Scale bar, 500 nm. ( d ) HRTEM image of ZnO. Scale bar, 5 nm. ( e , f ) FESEM image of CuO. Inset of the panel f shows the interior particles at the broken part. Scale bars, 1 μm and 100 nm; e and f , respectively. ( g ) TEM image of CuO. Scale bar, 500 nm. ( h ) HRTEM image of CuO. Scale bar, 5 nm. SAED patterns (insets of TEM images) show the single-crystal diffraction. Full size image To investigate the mechanism for the formation of the mesocrystals, we compared the powder X-ray diffraction (XRD) patterns ( Supplementary Fig. 5 ) and FESEM images ( Supplementary Figs 6–9 ) of the products obtained at various synthesis temperatures. For the ZnO mesocrystals ( Supplementary Fig. 5a ), the polymer-assisted growth of Zn(OH) (NO 3 )·H 2 O crystals started at 250 °C during the evaporation of water, along with the simultaneous production of NH 4 NO 3 crystals ( Supplementary Fig. 6a ), as described by equation (1) When the annealing temperature was increased to 300 °C, the polymer was removed ( Supplementary Fig. 6b ), and Zn(OH)(NO 3 )·H 2 O topotactically transformed into pure ZnO ( Supplementary Fig. 5a ) by equation (2) [27] , [28] For the CuO mesocrystals ( Supplementary Fig. 5b ), the intermediate crystal Cu 2 (OH) 3 NO 3 appeared at 200 °C. The transformation of the intermediate crystals into CuO is very similar to that of the intermediate crystal into ZnO ( Supplementary Fig. 7 ), and the reaction processes are summarized by equations (3) and (4) [29] , [30] Structure of nanocomposite mesocrystals Our approach has laid the foundation for further synthesis of nanocomposite mesocrystal materials consisting of two different metal oxide nanocrystals. For example, zinc and copper nitrates with different ratios were used as metal precursors to synthesize nanocomposite mesocrystals consisting of ZnO and CuO (ZnO-CuO) ( Fig. 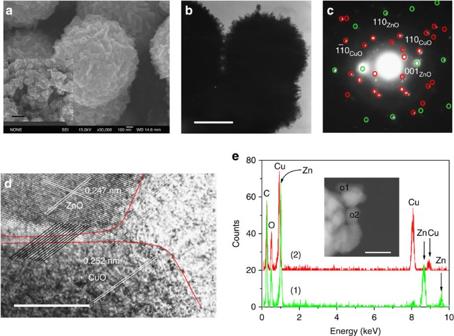Figure 2: Nanocomposite mesocrystals. (a) FESEM image. The inset shows the interior particles at the broken part. Scale bars, 100 nm. (b) TEM image. Scale bar, 500 nm. (c) SAED pattern. The green and red circles represent the spots corresponding to ZnO and CuO, respectively. (d) HRTEM image of ZnO-CuO mesocrystal. Scale bar, 10 nm. (e) EDX point spectra (1) and (2) taken at positions (o1) and (o2) indicated on the HAADF-STEM image (inset) of nanoparticles on the edge of the ZnO-CuO mesocrystal. Scale bar, 50 nm. 2 and Supplementary Table 2 ). The two metal precursors were mixed in aqueous solutions containing the additives P123 and NH 4 NO 3 . When the annealing temperature reaches 200 °C, the intermediate crystal obtained is a composite of Zn(OH)NO 3 ·H 2 O and Cu 2 (OH) 3 (NO 3 ) ( Supplementary Fig. 8 ). Porous mesocrystal structures were obtained by further annealing the intermediate crystals at 250 °C. Figure 2: Nanocomposite mesocrystals. ( a ) FESEM image. The inset shows the interior particles at the broken part. Scale bars, 100 nm. ( b ) TEM image. Scale bar, 500 nm. ( c ) SAED pattern. The green and red circles represent the spots corresponding to ZnO and CuO, respectively. ( d ) HRTEM image of ZnO-CuO mesocrystal. Scale bar, 10 nm. ( e ) EDX point spectra (1) and (2) taken at positions (o1) and (o2) indicated on the HAADF-STEM image (inset) of nanoparticles on the edge of the ZnO-CuO mesocrystal. Scale bar, 50 nm. Full size image The XRD peaks of the mesocrystals are consistent with those known to be associated with the crystal structures of the ZnO and CuO phases ( Supplementary Fig. 9 , JCPDF #65-3,411 for ZnO and JCPDF #48-1,548 for CuO). Thermogravimetric analysis of the as-synthesized ZnO-CuO mesocrystal in air showed a weight loss of 0.25% between 200 and 350 °C owing to the removal of residual P123 ( Supplementary Fig. 10 ). We also measured Fourier transform infrared spectrum of the ZnO-CuO mesocrystal ( Supplementary Fig. 11 ). The characteristic peaks of P123 were not observed, thus suggesting that P123 was almost completely removed by annealing at 500 °C for 2 h. Figure 2a and b , respectively, show FESEM and TEM images of a ZnO(0.4)-CuO(1.0) mesocrystal (Zn:Cu molar ratio of 0.4:1.0, which was determined by inductively coupled plasma atomic emission spectroscopy analysis ( Supplementary Table 2 )) with a spherical structure and a size of about 1 μm assembled from small nanoparticles. The results of ZnO-CuO mesocrystals with different compositions (Zn:Cu molar ratios of 1.0:1.0 and 1.4:1.0) are given in Supplementary Figs 12 and 13 . The specific surface area of the ZnO-CuO mesocrystal is 3.6 m 2 g −1 , and the pore diameter has a broad distribution with an average of 54 nm ( Supplementary Fig. 14 ). The SAED pattern for one particle is consistent with the single-crystalline structures of both the ZnO and CuO phases ( Fig. 2c ). The HRTEM images taken at the surface region of the mesocrystal showed that the ZnO and CuO phases have similar crystalline lattices in the same crystallographic directions across the ZnO and CuO nanocrystals, with consistent lattice fringes ( Fig. 2d ). The energy-dispersive X-ray spectroscopy (EDX) point spectra shown in Fig. 2e suggest that position 1 is on a ZnO particle and position 2 is on a CuO particle. It can be estimated that the nanocrystal sizes of ZnO and CuO are 37±10 and 26±10 nm, respectively, which are consistent with the XRD results ( Supplementary Table 1 ). X-ray photoelectron spectroscopy (XPS) spectra further demonstrated that all the surface Zn species in the ZnO-CuO mesocrystal were present in the form of ZnO (ref. 31 ), which has a binding energy of 1,021.4 eV in the Zn 2 p 3/2 spectrum ( Supplementary Fig. 15 ). This binding energy value is exactly the same as that obtained from a pure ZnO mesocrystal. In addition, the presence of ZnO nanocrystals embedded in the CuO framework had no significant influence on the Cu 2 p XPS spectra [31] . Thus, the ZnO was present mainly as a separate phase in the ZnO-CuO mesocrystal. HAADF-STEM-EDX measurements of nanocomposite mesocrystals The high-angle annular dark-field (HAADF)-scanning TEM (STEM)-EDX line scan results clearly illustrate the distribution of ZnO and CuO nanocrystals on the surface of a single ZnO(0.4)-CuO(1.0) mesocrystal sphere ( Fig. 3a–c ). The EDX pattern ( Fig. 3b ) reveals that the molar content of ZnO is about 36% on the surface. As seen from Fig. 3c , the signal intensity patterns of Zn and Cu are different. The peaks in the Zn profile are probably indicative of the ZnO nanocrystals on the surface, whereas the Cu profile is more flat because of the higher abundance of CuO. The intersections of the two profiles are assigned as interfaces between ZnO and CuO nanocrystals. To investigate the internal distribution of ZnO and CuO nanocrystals in the ZnO-CuO mesocrystal, the mesocrystals were sectioned by an ultramicrotome to reveal their cross-sections. 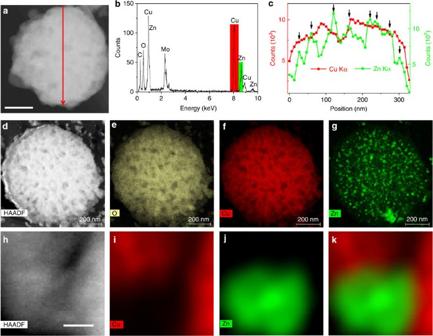Figure 3: ZnO-CuO mesocrystal structural characterization. (a) HAADF-STEM image of a ZnO-CuO mesocrystal. Scale bar, 100 nm. (b) EDX spectrum of ZnO-CuO mesocrystal (the Kα peaks of Cu (8.04 keV) and Zn (8.63 keV) are highlighted in red and green, respectively). (c) EDX line scan profile across the single ZnO-CuO mesocrystal along the red line in imagea. The arrows indicate the ZnO nanocrystals on the mesocrystal surface. (d) Cross-sectional HAADF-STEM image of a ZnO-CuO mesocrystal. Scale bar, 200 nm. (e–g) EDX elemental mapping of O, Cu and Zn in the cross-section of a ZnO-CuO mesocrystal. (h) High-resolution cross-sectional HAADF-STEM image. Scale bar, 10 nm. (i,j) High-resolution EDX elemental mapping of Zn and Cu in the cross-section of a ZnO-CuO mesocrystal. (k) Merged image ofiandj. Figure 3d gives the cross-sectional HAADF-STEM image. There are many pores with different sizes inside the ZnO-CuO mesocrystal, inferring that the mesocrystal is assembled by small nanoparticles. The internal composition of the ZnO-CuO mesocrystal was further investigated by HAADF-STEM-EDX elemental mapping analyses, which revealed the nanoscale elemental composition as well as the spatial uniformity of the element distribution in the ZnO-CuO mesocrystal ( Fig. 3e–g ). The EDX elemental mapping results clearly show that Cu and O are homogeneously distributed over the mesocrystal ( Fig. 3e,f ), while the Zn is detected as punctate dots dispersed over the whole mesocrystal ( Fig. 3g ). The concentration of the Zn elements tends to increase with increasing composition of ZnO in the ZnO-CuO mesocrystal ( Supplementary Figs 12e and 13e ). Moreover, a high-resolution HAADF-STEM-EDX-mapping analysis visualizes that ZnO and CuO nanocrystals inside the mesocrystal are in physical contact with each other; this would facilitate the electronic communication between them ( Fig. 3h–k ) [7] . Figure 3: ZnO-CuO mesocrystal structural characterization. ( a ) HAADF-STEM image of a ZnO-CuO mesocrystal. Scale bar, 100 nm. ( b ) EDX spectrum of ZnO-CuO mesocrystal (the Kα peaks of Cu (8.04 keV) and Zn (8.63 keV) are highlighted in red and green, respectively). ( c ) EDX line scan profile across the single ZnO-CuO mesocrystal along the red line in image a . The arrows indicate the ZnO nanocrystals on the mesocrystal surface. ( d ) Cross-sectional HAADF-STEM image of a ZnO-CuO mesocrystal. Scale bar, 200 nm. ( e – g ) EDX elemental mapping of O, Cu and Zn in the cross-section of a ZnO-CuO mesocrystal. ( h ) High-resolution cross-sectional HAADF-STEM image. Scale bar, 10 nm. ( i , j ) High-resolution EDX elemental mapping of Zn and Cu in the cross-section of a ZnO-CuO mesocrystal. ( k ) Merged image of i and j . Full size image PL property of mesocrystals To investigate the interfacial charge transfer in the ZnO-CuO mesocrystals, we first performed single-particle confocal fluorescence spectroscopy measurements [32] . 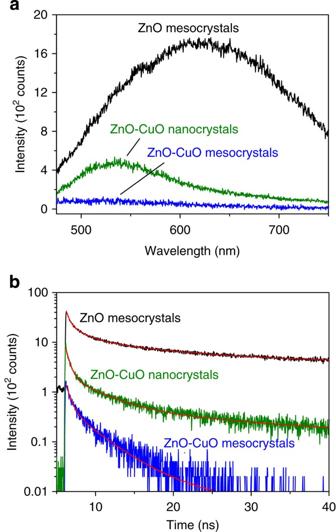Figure 4: Single-particle PL measurements. (a) Emission spectra and (b) decay profiles observed for ZnO mesocrystals (black), ZnO-CuO mesocrystals (blue) and ZnO-CuO nanocrystals (green). The red lines are the fitting lines. Figure 4a,b shows the photoluminescence (PL) spectra and decays of the mesocrystals on a quartz glass under 365 nm laser irradiation in ambient air (see Supplementary Fig. 16 for optical transmission and emission images). According to the literature [33] , the broad emission band at around 450–800 nm originates from defect-mediated charge recombination on the ZnO surface. The intensity-weighted average lifetime (‹ τ PL ›) for ZnO was 27 ns (‹ τ PL ›=25~30 ns for five different mesocrystals) ( Supplementary Table 3 ). After it was combined with CuO, however, this PL was strongly quenched (see Fig. 4a,b and Supplementary Fig. 16b ) and ‹ τ PL › was reduced to 2.7 ns (‹ τ PL ›=1.5~3.5 ns for five different mesocrystals) ( Supplementary Table 3 ). The average reaction rate is roughly calculated to be 3.3 × 10 8 s −1 from ‹ τ PL ZnO-CuO › −1 −‹ τ PL ZnO › −1 , where ‹ τ PL ZnO-CuO › and ‹ τ PL ZnO › are the average PL lifetimes for the ZnO-CuO and ZnO mesocrystals, respectively. To demonstrate the superiority of the superstructure, a composite of ZnO and CuO nanocrystals (ZnO-CuO nanocrystals) was prepared by the same procedure without adding P123 (the molar ratios of this sample are the same as those in the composite mesocrystal; Supplementary Fig. 17 ) and used as a reference. The ‹ τ PL › value obtained for the ZnO-CuO nanocrystals was 16 ns (‹ τ PL ›=9~19 ns for five different locations; Supplementary Fig. 16d and Supplementary Table 3 ), thus suggesting that efficient charge transfer occurred within the composite mesocrystals. Figure 4: Single-particle PL measurements. ( a ) Emission spectra and ( b ) decay profiles observed for ZnO mesocrystals (black), ZnO-CuO mesocrystals (blue) and ZnO-CuO nanocrystals (green). The red lines are the fitting lines. Full size image EPR spectra of mesocrystals Electron paramagnetic resonance (EPR) spectroscopy was further employed to monitor-native defects in the ZnO-CuO mesocrystals and their photoresponse. 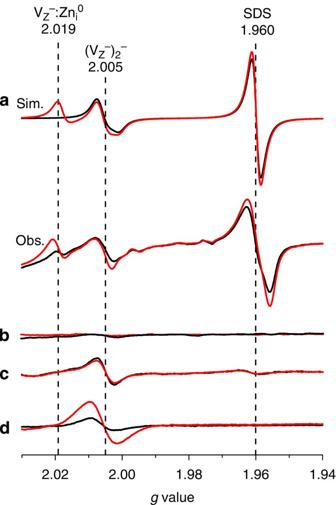Figure 5: EPR spectroscopy measurements. EPR spectra of (a) ZnO mesocrystals, (b) CuO mesocrystals, (c) ZnO-CuO mesocrystals and (d) ZnO-CuO nanocrystals at 77 K in vacuum (black lines are acquired in dark and red lines are under ultraviolet irradiation; sim. and obs. are the simulated and observed spectra, respectively). To reproduce the observed spectrum for ZnO, simulations were performed with the following EPR parameters:g=1.960,g=2.005 (gxx=2.0077,gyy=2.0010,gzz=2.0059) andg=2.019 (gxx=2.0185,gyy=2.0188,gzz=2.0044)34,35. Figure 5a shows the EPR spectrum of ZnO mesocrystals recorded at 77 K in a vacuum. Both the observed and simulated EPR spectra exhibit intense sharp resonance signals at g =1.960 and g =2.005 in the absence of ultraviolet light (black lines). The resonance signal at g =1.960 has been assigned to shallow donor states due to impurities or defects in the ZnO (possibly singly ionized oxygen vacancies ( V O + )) [34] , [35] . The resonance signal at g =2.005 has been attributed to two mutually close zinc vacancies with one hole (( V Z − ) 2 − ) [34] , [35] . After ultraviolet light irradiation (red lines), a new resonance signal at g =2.019 from a zinc vacancy with a hole has been observed [34] , [35] , which indicates the formation of photogenerated charges localized on one of the four oxygen ions, V Z − , and an internode neutral zinc atom Zn i 0 ( V Z − :Zn i 0 ). In the case of CuO mesocrystals, no such EPR signals are observed in the absence of ultraviolet light or under ultraviolet light ( Fig. 5b ). When ZnO is combined with CuO to form p – n composite mesocrystals, the EPR resonance signal only appeared at g =2.005 with or without ultraviolet light irradiation ( Fig. 5c ). On the other hand, the ZnO-CuO nanocrystals exhibit an intense resonance peak at g =2.005 after the ultraviolet light irradiation, indicating the formation of ( V Z − ) 2 − ( Fig. 5d ). Figure 5: EPR spectroscopy measurements. EPR spectra of ( a ) ZnO mesocrystals, ( b ) CuO mesocrystals, ( c ) ZnO-CuO mesocrystals and ( d ) ZnO-CuO nanocrystals at 77 K in vacuum (black lines are acquired in dark and red lines are under ultraviolet irradiation; sim. and obs. are the simulated and observed spectra, respectively). To reproduce the observed spectrum for ZnO, simulations were performed with the following EPR parameters: g =1.960, g =2.005 ( g xx =2.0077, g yy =2.0010, g zz =2.0059) and g =2.019 ( g xx =2.0185, g yy =2.0188, g zz =2.0044) [34] , [35] . Full size image Time-resolved diffuse reflectance spectra of mesocrystals To clarify the ultrafast interfacial charge transfer dynamics, we conducted femtosecond time-resolved diffuse reflectance spectroscopy measurements. Immediately after the 330-nm laser excitation of the ZnO mesocrystal sample, a broad absorption band appeared in the near-infrared wavelength region ( Fig. 6a ). The observed absorption spectrum is considered to be superimposed with those of the trapped electrons and free electrons (increasing monotonically from the visible to near-infrared regions) in ZnO (ref. 36 ). A similar observation has been reported for TiO 2 nanoparticles [37] . For a time period of 0.4–100 ps, the concentration of the electrons decreased in a multi-exponential fashion owing to the charge recombination of these electrons with the holes ( Fig. 6e ). In the case of CuO mesocrystal, most of the transient absorption at around 900–1,200 nm decays on a subpicosecond timescale, suggesting either rapid surface trapping or recombination of photogenerated charges ( Fig. 6b ). Long-lived species with an absorption peak at ~900 nm are presumably the deeply trapped charges. Both ZnO(0.4)-CuO(1.0) mesocrystal ( Fig. 6c ) and nanocrystal ( Fig. 6d ) samples showed similar broad absorption spectra immediately after the laser flash, while their decay kinetics are obviously different ( Fig. 6e ). The decay times measured at 1,100 nm are 0.43 ps (90%) and 11 ps (10%) for mesocrystals and 1.1 ps (81%) and 16 ps (19%) for nanocrystals ( Supplementary Table 4 ). Furthermore, the transient absorption spectrum of ZnO-CuO mesocrystal probed at 100 ps exhibits the accumulation of CuO charges in the mesocrystals ( Fig. 6c ). 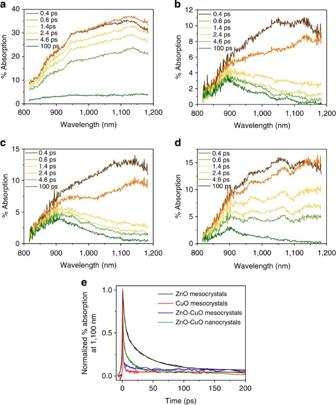Figure 6: Time-resolved diffuse reflectance spectroscopy measurements. Transient absorption spectra of (a) ZnO mesocrystals, (b) CuO mesocrystals, (c) ZnO-CuO mesocrystals and (d) ZnO-CuO nanocrystals. (e) Time traces observed at 1,100 nm. The bold and fine lines represent the experimental data and the fitting results, respectively. Figure 6: Time-resolved diffuse reflectance spectroscopy measurements. Transient absorption spectra of ( a ) ZnO mesocrystals, ( b ) CuO mesocrystals, ( c ) ZnO-CuO mesocrystals and ( d ) ZnO-CuO nanocrystals. ( e ) Time traces observed at 1,100 nm. The bold and fine lines represent the experimental data and the fitting results, respectively. Full size image On the basis of the above results, we summarize the general method as follows ( Fig. 7 ). As the annealing temperature gradually increases, seed nanoparticles stabilized by P123 polymers self-assemble and undergo attachment to form intermediate crystals with specific morphologies. P123 is known to be an amphiphilic surfactant capable of forming micelles to aid in the growth of metal oxide nanocrystals [38] , [39] . The appropriate ratio of metal ions to nitrate ions is believed to control the structure and composition of the intermediate crystals. The intermediate crystals then topotactically transform into metal oxide mesocrystals while maintaining their single-crystalline structures in the last step. 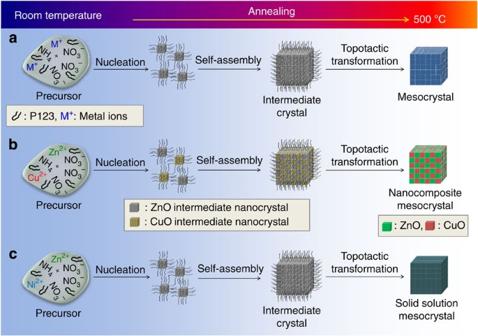Figure 7: Proposed formation mechanisms of metal oxide mesocrystals. (a) Metal oxide mesocrystals consisting of a single-metal element (for example, ZnO, CuO, NiO and TiO2). (b) Nanocomposite mesocrystals. (c) Solid solution mesocrystals. Figure 7: Proposed formation mechanisms of metal oxide mesocrystals. ( a ) Metal oxide mesocrystals consisting of a single-metal element (for example, ZnO, CuO, NiO and TiO 2 ). ( b ) Nanocomposite mesocrystals. ( c ) Solid solution mesocrystals. Full size image To gain an insight into the formation mechanism of mesocrystals, the intermediate crystals and P123 were separated by extraction with water and dichloromethane, respectively, after heating of the precursor solution at 100 °C for 1 h. In situ dynamic light scattering (DLS) experiments revealed that intermediate nanoparticle aggregates form when the heating temperature reaches 60 °C ( Supplementary Fig. 18 ). As shown in Supplementary Fig. 19 , the isolated materials are microspheres (0.5–1 μm size) containing Zn and Cu elements at the 0.4:1.0 molar ratio and consist of assembled nanoparticles. Thus, all the experimental results confirm the validity of the proposed mechanisms in Fig. 7b . When zinc and nickel nitrates were chosen as precursors ( Fig. 7c ), the crystalline structure of the resulting material was a solid solution of Zn 0.2 Ni 0.8 O ( Supplementary Fig. 20 ). This substitution causes a small shift in the XRD peaks ( Supplementary Fig. 21 ) [40] . Although the ionic radius of Zn 2+ (0.074 nm) is more similar as Cu 2+ (0.073 nm), compared with Ni 2+ (0.069 nm), a solid solution of ZnO and CuO was not obtained under the synthesis conditions studied here. This is mainly because of the larger difference of Zn 2+ and Cu 2+ coordination environment in ZnO and CuO. The Zn 2+ ions in ZnO prefer tetrahedral coordination, while Cu 2+ ions in CuO are in Jahn–Teller-distorted octahedral coordination [41] , [42] . These different coordination environments result in the low degree of solid-state solubility between CuO and ZnO. In contrast, the coordination environment of the Zn 2+ sites in ZnO is suitable for Ni 2+ (refs 42 , 43 ). This is the reason why CuO and ZnO are phase separate, while NiO and ZnO form a solid solution. Nanocomposites exhibit numerous unique properties and have potential uses in a wide range of applications. For instance, the photoinduced charge transfer between different semiconductors is very important for photocatalysis and optoelectronic applications [18] , [19] . ZnO is a typical n -type semiconductor, and CuO is an important p -type semiconductor [44] , [45] . The energy diagram presented in Supplementary Fig. 22 suggests that photogenerated electrons and holes in ZnO can be transferred to the conduction band and valance band of CuO, respectively. A basically similar mechanism has been proposed for charge transfer between TiO 2 and CuO (refs 46 , 47 ). Thus, as shown in Fig. 4 , the ZnO PL was significantly quenched due to the efficient interfacial charge transfer occurring between ZnO and CuO because of the intimate contact between adjacent nanocrystals in the mesocrystal. This conclusion was further supported by the results of EPR ( Fig. 5 ) and time-resolved diffuse reflectance ( Fig. 6 ) measurements. In summary, we described a facile and general topotactic transformation approach to the synthesis of pure metal oxide mesocrystals. NH 4 NO 3 and P123 were used as additives to control the self-assembly and attachment of nanoparticles to form intermediate crystals with specific compositions and morphologies. Other surfactants (like CTAB and F127) [48] , copolymers [49] , non-ionic polymers (such as PVP) [50] and functionalized polymers [51] might also be used as organic additives to form mesocrystals. Furthermore, for the first time, we synthesized a nanocomposite by simply mixing different metal precursors. Such nanocomposite mesocrystalline heterostructures facilitate the charge transfer between p - and n -type semiconductors, which is beneficial for applications in many fields such as photovoltaics and photocatalysis. Preparation of metal oxide mesocrystals ZnO mesocrystals were prepared from a precursor solution of Zn(NO 3 ) 2 (Wako), H 2 O, NH 4 NO 3 (Wako) and P123 (Aldrich, amphiphilic triblock copolymer polyethylene oxide/poly( p -phenylene oxide)/polyethylene oxide ((EO) 20 (PO) 70 (EO) 20 )) (molar ratio=123:32,000:444:1). CuO mesocrystals were prepared from a precursor solution of Cu(NO 3 ) 2 (Wako), H 2 O, NH 4 NO 3 and P123 (molar ratio=39:29,300:444:1). ZnO-CuO mesocrystals were prepared from a precursor solution of Zn(NO 3 ) 2 , Cu(NO 3 ) 2 , H 2 O, NH 4 NO 3 and P123 (for example, molar ratio=15:32:29,800:444:1 for ZnO(0.4)-CuO(1.0) mesocrystals). The above precursors (10 ml) were placed on a glass bottles 3.5 cm (diameter) × 7.8 cm (height). The precursor was calcined in air using a heating rate of 10 °C min −1 at 500 °C for 2 h. Structural characterizations The samples were characterized using XRD (Rigaku, Smartlab at 40 kV and 200 mA, Cu Kα source), FESEM (JEOL, JSM-6330FT), TEM (JEOL, JEM 3000F, operated at 300 kV or Hitachi H-800, operated at 200 kV), HAADF-STEM-EDX (FEI, Tecnai G2, operated at 120 kV or Tecnai Osiris, operated at 200 kV), inductively coupled plasma atomic emission spectroscopy (Perkin Elmer, Optima 3000 XL), DLS (Otsuka Electronics, ELSZ-1000), thermogravimetric analysis (Rigaku, Thermo plus EVO II/TG-DTA (TG8120)), Fourier transform infrared (JASCO, FT/IR-4100), XPS (ULVACPHI-PHI, Quantera SXM) and nitrogen sorption (BEL Japan, BEL-SORP max). A Leica Ultracut EM UC6 ultramicrotome was used for making cross-section samples with a thickness of ~100 nm. The Brunauer–Emmett–Teller method was utilized to calculate the specific surface area. The pore volume and pore diameter distribution were derived from the adsorption isotherms by the Barrett–Joyner–Halenda model. Single-particle fluorescence spectroscopy measurements The PL from individual mesocrystals was recorded using an objective-scanning confocal microscope system (PicoQuant, MicroTime 200) coupled with an Olympus IX71 inverted fluorescence microscope. The samples spin coated on the cleaned quartz coverslips were excited through an oil objective (Olympus, UPLSAPO 100XO; 1.40 numerical aperture, × 100) with a circular-polarized 365-nm pulsed laser (Spectra-Physics, Mai TAi HTS-W with an automated frequency doubler, Inspire Blue FAST-W; 0.8 MHz repetition rate) controlled by a PDL-800B driver (PicoQuant). The instrument response function of ~100 ps was obtained by measuring the scattered laser light to analyse the temporal profile. The emission was collected with the same objective and detected by a single-photon avalanche photodiode (Micro Photon Devices, PDM 50CT) through a dichroic beam splitter (Chroma, z405rdc), long-pass filter (Chroma, HQ435LP) and 50 μm pinhole for spatial filtering to reject out-of-focus signals. The data collected using the PicoHarp 300 TCSPC module (PicoQuant) were stored in the time-tagged time-resolved mode, recording every detected photon with its individual timing. All of the experimental data were obtained at room temperature. EPR spectroscopy measurements X-band EPR spectra were recorded on a JEOL JES-RE2X electron spin resonance spectrometer at 77 K. EPR spectra of the samples were taken before and after ultraviolet light irradiation (Asahi Spectra, REX-250) at 77 K. The g values were calibrated using 2,2-diphenyl-1-picryl-hydrazil ( g =2.0036) as a standard. Time-resolved diffuse reflectance spectroscopy measurements The femtosecond diffuse reflectance spectra were measured by the pump and probe method using a regeneratively amplified titanium sapphire laser (Spectra-Physics, Spitfire Pro F, 1 kHz) pumped by a Nd:YLF laser (Spectra-Physics, Empower 15). The seed pulse was generated by a titanium sapphire laser (Spectra-Physics, Mai Tai VFSJ-W; fwhm 80 fs). The fourth harmonic generation (330 nm, 3 mJ pulse −1 ) of the optical parametric amplifier (Spectra-Physics, OPA-800CF-1) was used as the excitation pulse. A white light continuum pulse, which was generated by focusing the residual of the fundamental light on a sapphire crystal after the computer-controlled optical delay, was divided into two parts and used as the probe and the reference lights, of which the latter was used to compensate the laser fluctuation. Both probe and reference lights were directed to the sample powder coated on the glass substrate, and the reflected lights were detected by a linear InGaAs array detector equipped with the polychromator (Solar, MS3504). The pump pulse was chopped by the mechanical chopper synchronized to one-half of the laser repetition rate, resulting in a pair of spectra with and without the pump, from which the absorption change (% absorption) induced by the pump pulse was estimated. All measurements were carried out at room temperature. How to cite this article: Bian, Z. et al. A nanocomposite superstructure of metal oxides with effective charge transfer interfaces. Nat. Commun. 5:3038 doi: 10.1038/ncomms4038 (2014).